Hydride-based antiperovskites with soft anionic sublattices as fast alkali ionic conductors Most solid-state materials are composed of p-block anions, only in recent years the introduction of hydride anions (1s 2 ) in oxides (e.g., SrVO 2 H, BaTi(O,H) 3 ) has allowed the discovery of various interesting properties. Here we exploit the large polarizability of hydride anions (H – ) together with chalcogenide (Ch 2– ) anions to construct a family of antiperovskites with soft anionic sublattices. The M 3 HCh antiperovskites (M = Li, Na) adopt the ideal cubic structure except orthorhombic Na 3 HS, despite the large variation in sizes of M and Ch. This unconventional robustness of cubic phase mainly originates from the large size-flexibility of the H – anion. Theoretical and experimental studies reveal low migration barriers for Li + /Na + transport and high ionic conductivity, possibly promoted by a soft phonon mode associated with the rotational motion of HM 6 octahedra in their cubic forms. Aliovalent substitution to create vacancies has further enhanced ionic conductivities of this series of antiperovskites, resulting in Na 2.9 H(Se 0.9 I 0.1 ) achieving a high conductivity of ~1 × 10 –4 S/cm (100 °C). Perovskites with a formula of ABX 3 (A, B: cations, X: anions) are ubiquitous and central to electronics, photonics, and energy technologies [1] , [2] . Their electronically inverted analogs, antiperovskites, are playing an increasingly major role in solid-state chemistry and physics owing to their various intriguing properties, such as giant magnetoresistance in Mn 3 GaC [3] , superconductivity in Ni 3 MgC [4] , negative thermal expansion in Mn 3 BA (B = Zn, Cu etc. ; A = N, C) [5] , [6] , efficient water splitting electrocatalytic activity in Ni 3 FeN [7] , superionic conductivity in Ag 3 SI [8] and large capacity in (Li 2 Fe)OCh (Ch = S, Se, Te) as lithium battery cathodes [9] . In particular, lithium-rich and sodium-rich antiperovskites (LiRAPs and NaRAPs), for example, M 3 OCl, M 3 OBr (M = Li, Na), and Na 3 OBH 4 , have recently attracted a great deal of attention as they exhibit a high lithium (or sodium) ionic conductivity and are thus regarded as promising solid-state electrolytes enabling high-energy-density lithium metal batteries [10] , [11] , [12] , [13] . Similar to the F – superionic conductivity in NaMgF 3 perovskite [14] , the antiperovskite M 3 OCl allows Li + /Na + superionic conductivity benefited from the M-rich content (60 at% in Li 3 OCl) [10] , [13] . Another advantage of antiperovskite is its extraordinary chemical diversity. Similar to perovskite, a variety of combinations of elements can be accommodated, while maintaining the simple structural topology, thereby offering an ideal situation to easily and fully characterize fast ionic transport [15] , [16] . A very recent study on Li 3 OCl indicated that the presence of hydroxide (OH – ), providing the composition of Li 3– x O 1– x (OH) x Cl, or ultimately Li 2 (OH)Cl [17] . In the search of new fast ion-conducting solid-state materials [18] , [19] , [20] , [21] , [22] , [23] , [24] , [25] , [26] , [27] , a great deal of effort has been made to understand ionic transport in Li-ion conductors, where two features of the anion-host matrix have been highlighted [18] , [19] , [20] . The first feature proposed by Ceder et al. is that the anion arrangement of body-centered cubic (bcc) provides the lowest migration barrier for Li-ion diffusion, rather than a close-packed (fcc or hcp) anion framework [27] . Antiperovskites host the bcc framework composed of A- and B-site anions [10] , [13] , [16] . The second feature is that polarizable anions can critically soften and flatten the cationic transport landscape, leading to lower activation energy and higher ionic conductivity [23] , [25] , [28] , [29] , [30] , [31] . In fact, thiophosphate ionic conductors, such as Li 10 GeP 2 S 12 with the highest Li-ion conductivity, are believed to benefit from a soft and polarizable anion lattice [32] . In this study, we present the synthesis of a series of LiRAPs and NaRAPs, M 3 HCh (M = Li, Na; Ch = S, Se, Te) with both anionic sites occupied by soft and polarizable anions of H – and Ch 2– (Fig. 1 ) [33] , [34] . To our knowledge, LiRAPs and NaRAPs have been obtained only with oxide/hydroxide anions at the B site, which considerably limits the scope of structures and properties. Experimental and theoretical investigations have revealed that the occupation of highly polarizable and size-flexible H – anions at the B site in M 3 HCh introduces several interesting features, including the stability and robustness of the ideal cubic structure and softening of phonon mode associated with HM 6 octahedral rotation, which could be advantageous for realizing high Li + /Na + conductivity. The energy migration barriers based on vacancy and interstitial dumbbell mechanisms are found to be lower than those of oxide-based LiRAPs and NaRAPs. Li + /Na + vacancy creation via iodine (I – ) doping (for Ch 2– ) is a potential strategy to increase the ionic conductivity of this series of antiperovskites, where I-doped cubic Na 3 HSe with formula Na 2.9 H(Se 0.9 I 0.1 ) delivers a high total Na + conductivity exceeding 1 × 10 –4 S/cm at 100 °C with a low bulk activation energy of ~0.18 eV in agreement with the calculated one (~0.16 eV). Fig. 1: Crystal structure of hydride-based M 3 HCh antiperovskite (M = Li, Na). a Crystal structure of the cubic antiperovskite (space group Pm–3 m ). In this study, we obtained Li 3 HCh (Ch = S, Se, Te) and Na 3 HCh (Ch = Se, Te), where H – anion (blue; B site) is bonded with Li + /Na + cations (green) forming HLi 6 /HNa 6 octahedron, while chalcogenide anion (yellow; A site) sits in cuboctahedral coordination site. As opposed to conventional perovskites, the cubic structure is robust in a wide range of compositions. b The orthorhombic anti-GdFeO 3 type (space group Pnma ) Na 3 HS with HNa 6 octahedral tilting. Full size image Structure determination The high-resolution synchrotron X-ray diffraction (SXRD) pattern of the sample prepared using LiH and Li 2 S at 5 GPa and 700 °C (Fig. 2a ) shows the formation of a highly crystalline compound, along with impurity phases that could be identified as LiH, Li 2 S, and BN (insulating high-pressure sleeve). The diffraction profile of the main phase was indexed in a cubic system with the lattice parameter of a = 3.85189(6) Å (see Supplementary Fig. 1 ), which is comparable to those of reported antiperovskite oxyhalides Li 3 OCl and Li 3 OBr ( a = 3.900 Å and 3.989 Å, respectively) with the space group Pm–3m [10] , [12] . Fig. 2: Structural determination of Li 3 HS. Rietveld refinement of a SXRD and b ND. The red crosses, black solid line, blue solid line, and green dashes denote, respectively, the observed, calculated, difference intensities, and calculated Bragg reflections (from top to bottom: Li 3 HS, Li 2 S, LiH, BN in a ; Li 3 HS, LiH in b ). Full size image Given the known antiperovskites, e.g., Ag 3 SI [8] , Li 3 OCl [10] , with a smaller anion at the octahedral B site and a larger one at the cuboctahedral A site, we performed Rietveld refinement assuming S 2– at the 1 b (1/2, 1/2, 1/2) Wyckoff position and H – at the 1 a (0, 0, 0) site and Li + at the 3 d (1/2, 0, 0) site within the space group of Pm-3m , corresponding to a stoichiometric Li 3 HS formula. The Rietveld refinement converged successfully with values of R Bragg = 4.28% and R f = 2.87% (see Fig. 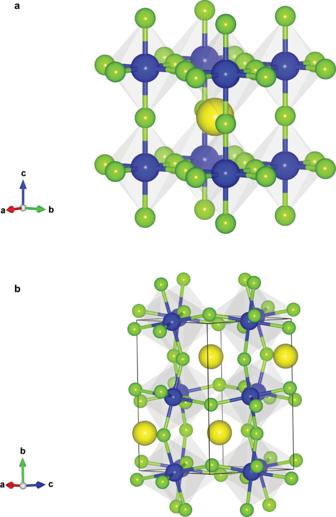Fig. 1: Crystal structure of hydride-based M3HCh antiperovskite (M = Li, Na). aCrystal structure of the cubic antiperovskite (space groupPm–3m). In this study, we obtained Li3HCh (Ch = S, Se, Te) and Na3HCh (Ch = Se, Te), where H–anion (blue; B site) is bonded with Li+/Na+cations (green) forming HLi6/HNa6octahedron, while chalcogenide anion (yellow; A site) sits in cuboctahedral coordination site. As opposed to conventional perovskites, the cubic structure is robust in a wide range of compositions.bThe orthorhombic anti-GdFeO3type (space groupPnma) Na3HS with HNa6octahedral tilting. 2a and Supplementary Table 1 ). Swapping the anionic octahedral B site and cubocathedral A site to give a Li 3 SH led to poor refinement values of R Bragg = 22.6% and R f = 11.2% (Supplementary Fig. 2 ). Subsequently, time-of-flight powder neutron diffraction (ND) data were analyzed to better characterize lighter elements of H and Li. The presence of hydrogen in the sample can be readily seen from Fig. 2b exhibiting a high background intensity. The neutron refinement assuming the Li 3 HS structure yielded R wp = 1.35% and R Bragg = 6.28% thus confirming this structural model. Details of the refinement are listed in Supplementary Table 1 . It is found that the Li + , H – , and S 2– ions fully occupy their respective crystallographic sites, confirming the stoichiometric composition. We also examined the possibility of antisite disorder between H – and S 2– ; the Rietveld refinement allowing intersite anion exchange (Supplementary Table 1 ) in the stoichiometric composition led to the full occupancy ( g ) of H – at the B site ( g B (H) = 1.015(5)) with R wp = 1.37% and R Bragg = 6.64%, which implies that the anions are perfectly ordered. Note that Pd 3 H 0.89 In also has hydrogen at the octahedral site [35] , but this material may not be classified as hydride, given the metallic nature of this material and the nearly identical electronegativity between H (2.2) and Pd (2.2) [33] . Attempts to synthesize Li 3 HS compound at a lower pressure (1 GPa/3 GPa; 700 °C) or under ambient pressure (700 °C for 12 h) using LiH and Li 2 S was unsuccessful (Supplementary Fig. 3 ), indicating the high-pressure metastability of this antiperovskite. Materials variety To our knowledge, Li 3 HS is the first LiRAP with hydride anions at the B site. Next, we attempted to extend the antiperovskite family by including sodium as well as other chalcogenides under high-pressure and high-temperature reactions. The XRD patterns of Li 3 HSe and Li 3 HTe (Supplementary Fig. 4 ) are similar to Li 3 HS, with Bragg reflections moving toward lower angles, as expected from increasing ionic radii of chalcogenide anions. The obtained cell parameters of the cubic unit cell are 3.9744(5) Å for Li 3 HSe and 4.2221(3) Å for Li 3 HTe. Regarding the sodium system, the SXRD profiles of Na 3 HSe (Supplementary Fig. 5 ) and Na 3 HTe (Supplementary Fig. 6 ) are compatible with the cubic symmetry ( Pm–3m ) with a = 4.55901(7) Å and a = 4.76349(2) Å, respectively. The larger cell parameters result from the difference in the cationic size (Na + : 1.02 Å vs . Li + : 0.76 Å) [36] . Rietveld refinements of Na 3 HSe and Na 3 HTe validated the cubic antiperovskite structure, with detailed structural information in Supplementary Tables 2 and 3 . To gain microscopic information on the crystal structure, we conducted 23 Na nuclear magnetic resonance (NMR) with/without magic-angle spinning (MAS) for Na 3 HSe. The spectra in Supplementary Fig. 7 were fitted as a second-order quadrupolar line shape of the central transition with a common set of C Q = 1.61 MHz and η = 0.04, where C Q , and η denote a quadrupole coupling constant and an asymmetry parameter, respectively. The 23 Na MAS NMR spectrum shows a single sharp peak at 24.2 ppm, which indicates that all sodium atoms are in the same environment, in accordance with the refinement result that no significant chemical disorder occurs in Na 3 HSe (Supplementary Fig. 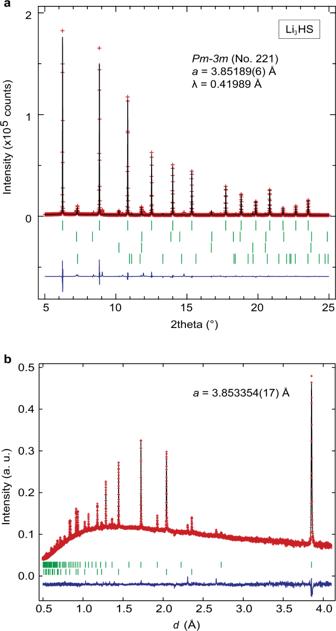Fig. 2: Structural determination of Li3HS. Rietveld refinement ofaSXRD andbND. The red crosses, black solid line, blue solid line, and green dashes denote, respectively, the observed, calculated, difference intensities, and calculated Bragg reflections (from top to bottom: Li3HS, Li2S, LiH, BN ina; Li3HS, LiH inb). 5 and Supplementary Table 2 ). This isotropic chemical shift (i.e., 24.2 ppm) is fairly consistent with that derived from DFT calculation (20.4 ppm with C Q = 1.95 MHz and ŋ DFT = 0). In the case of Na 3 HS, the XRD pattern (Supplementary Fig. 4 ) is clearly different and indexed by an orthorhombic unit cell ( a = 6.76037(9) Å, b = 8.89761(10) Å, and c = 6.28659(8) Å), which is related to the pristine cubic cell by √2 a p × 2 b p × √2 c p . This supercell and the extinct reflections suggest that Na 3 HS adopts an anti-GdFeO 3 structure ( Pnma space group, Fig. 1b ), as previously reported for M 3 OA (M = Sr, Eu, Ba, and A = Si, Ge) [37] . SXRD (Supplementary Fig. 8 ) and ND (Supplementary Fig. 9 ) data were refined assuming the anti-GdFeO 3 structure, yielding reasonable parameters, as listed in Supplementary Tables 4 and 5 . As shown in Fig. 3a , the normalized (cubic) lattice parameters of the LiRAP and NaRAP series both show linear dependence as a function of the chalcogen ionic radii, with approximately the same slope. As it is commonly done for normal perovskite structures, the tolerance factor ( t ) was estimated for our system, assuming the hydride ionic radius of 1.40 Å [36] , [38] . We found that the cubic structures are observed over a wide range 0.85 < t < 0.97 (Supplementary Table 6 ), in sharp contrast to perovskite oxides where slight deviations from unity readily lead to structural distortions. It is also noticed that oxide-based antiperovskites M 3 OA (M = Ca, Sr, Ba, Eu; A = Si, Ge, Sn, Pb) exhibit octahedral tilting when t < 0.97 [37] , implying that our hydride-based system is quite anomalous. The t value of the orthorhombic Na 3 HS is 0.84, slightly smaller than that of cubic Li 3 HS ( t = 0.85). 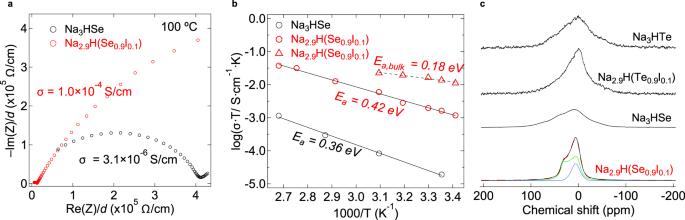Fig. 6: Na+diffusion in Na3HSe and Na2.9H(Se0.9I0.1). aImpedance plots at 100 °C of the cold-pressed pellets and the impedance is normalized to the respective pellet thickness.bArrhenius plots of the total conductivity (circles) and bulk conductivity (triangles).c23Na static NMR spectra measured under 7 T at room temperature. For Na2.9H(Se0.9I0.1), observed spectra (black solid), fitting spectra (red dashed), and deconvolved peak 1 withCQ= 1.30 MHz,ŋ= 0.16 (green) and peak 2 withCQ= 1.33 MHz,ŋ= 0.03 (blue). Fig. 3: Structural features of M 3 HCh antiperovskites (M = Li, Na). a Normalized (cubic) lattice parameters of M 3 HCh. For orthorhombic o-Na 3 HS, the cubic lattice parameter is an average of normalized lattice parameters. Lines are for the eye guidance. b The hydride anion (H – ) size obtained by subtracting M + radius from H – –M + bond length. Open triangles indicate the ionic radius of H – in hypothetical cubic c-Na 3 HS, which is calculated by using the average normalized cubic lattice parameter of the orthorhombic o-Na 3 HS. c BVS values for Ch 2– . Open triangles indicate the S 2– BVS for hypothetical cubic c-Na 3 HS. d Variation in bond length of B–M in BM 6 (B = H – , N 3– , O 2– , F – ) octahedra for M 3 BA antiperovskites and B–O in BO 6 (B = Fe 3+ , Cr 3+ , Zr 4+ ) octahedra for ABO 3 perovskites. The mentioned studies refer to Supplementary References (S1–S8). Full size image Phase stability Earlier studies on oxyhydrides have shown that the hydride anion (H – ) adapts itself to the different local environments, resulting in the hydride size flexibility; this unique feature brings about a number of novel properties such as high-pressure-induced coordination reversal in LaHO [33] , [39] , [40] , [41] , [42] . 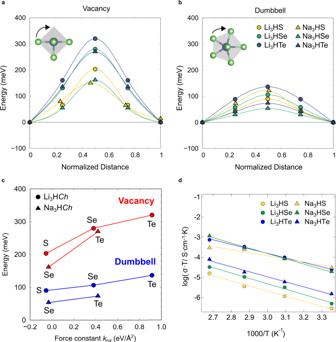This means that our assumption of the fixed hydride size (1.40 Å) for calculating the tolerance factor was not adequate. 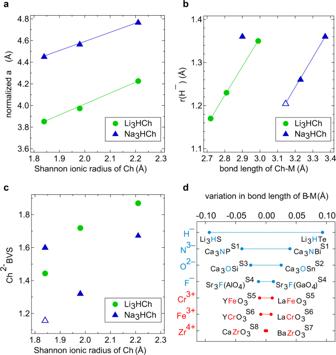Fig. 5: Ionic conductivities of M3HCh antiperovskites (M = Li, Na, and Ch = S, Se, Te). Low-barrier migration pathways foravacancy andbinterstitial dumbbell migration in M3HCh. Top-left insets show M+migration when viewing HM6octahedron from the top to down. For orthorhombic Na3HS, there are many migration pathways, one of which is shown as a representative example (see Supplementary Fig.15for details).cMigration barriers for cation transport via the vacancy and interstitial dumbbell mechanism in M3HCh as a function of the force constantkrotwith respect to the HM6rotational motion.dArrhenius plots of the total conductivity values for undoped M3HCh cold-pressed samples in the temperature range from 25 to 100 °C. 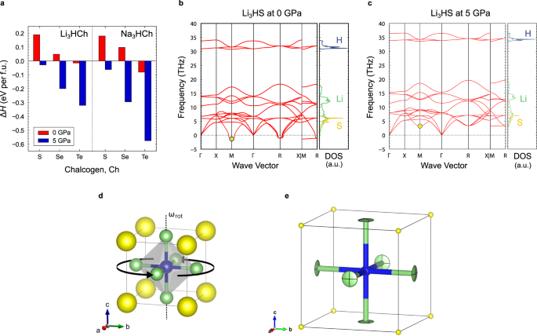Hence, we estimated the ionic radius of hydride anions, r(H – ) by subtracting the ionic radii of alkali metals, r(M + ) from the H–M bond lengths (a/2 in the case of the cubic system). Fig. 3: Structural features of M3HCh antiperovskites (M = Li, Na). aNormalized (cubic) lattice parameters of M3HCh. For orthorhombic o-Na3HS, the cubic lattice parameter is an average of normalized lattice parameters. Lines are for the eye guidance.bThe hydride anion (H–) size obtained by subtracting M+radius from H––M+bond length. Open triangles indicate the ionic radius of H–in hypothetical cubic c-Na3HS, which is calculated by using the average normalized cubic lattice parameter of the orthorhombic o-Na3HS.cBVS values for Ch2–. Open triangles indicate the S2–BVS for hypothetical cubic c-Na3HS.dVariation in bond length of B–M in BM6(B = H–, N3–, O2–, F–) octahedra for M3BA antiperovskites and B–O in BO6(B = Fe3+, Cr3+, Zr4+) octahedra for ABO3perovskites. The mentioned studies refer to Supplementary References (S1–S8). Fig. 4: Formation enthalpy and phonon calculations. aFormation enthalpy ΔHin the reaction MH + M2Ch → M3HCh (M = Li, Na) under 0 and 5 GPa.bPhonon band structures and partial phonon density of states (DOS) of Li, H, and S atoms in Li3HS under 0 GPa andc5 GPa. The negative number of the vertical axis represents imaginary frequency.dHM6octahedral rotation associated with the phonon mode denoted by yellow circles in phonon band dispersion, where ωrotis the frequency of the HM6rotational mode at M point.eDisplacement ellipsoids of Li atoms depicted at 50% probability level obtained from Rietveld refinement of ND in Li3HS. Figure 3b shows that the hydride substantially changes its size, with r(H – ) ranging from 1.17 Å to 1.36 Å. For the Li 3 HCh series, r(H – ) expands nearly linearly with the Ch–M bond length down the chalcogen group, in line with the increasing volume of HLi 6 octahedron and ChLi 12 cuboctahedron (Supplementary Fig. 10 ). A similar linear dependence can be recognized as long as the cubic phase of Na 3 HCh (including the hypothetical cubic c-Na 3 HS) is considered. Interestingly, the hydride size in the real orthorhombic o-Na 3 HS deviates from this linear relationship; r(H – ) in o-Na 3 HS greatly increases to the value closer to cubic Na 3 HTe. The particularly soft anion (H – ) with the flexible size is counterintuitive to the traditional hard-sphere model with fixed ionic radii when describing the bonding nature of ionic compounds. To better understand the swollen H – in orthorhombic o-Na 3 HS, we calculated bond valence sum (BVS) values of chalcogenide using the tabulated parameters [43] . Note that the size flexibility of hydride anion does not permit a reliable estimate of BVS for the hydride anion itself [40] . As shown in Fig. 3c , the BVS value for S 2– in hypothetical c-Na 3 HS is –1.16, which is unusually low, indicating that S 2– is greatly underbonded in the cuboctahedral site. Here, the flexible hydride comes into play. In o-Na 3 HS, the HNa 6 octahedron (due to swollen H – ) is greatly expanded (as displayed in Supplementary Fig. 10), which in turn reduces the SNa 12 volume and allows S 2– to gain an acceptable BVS value of –1.60. For the Li 3 HCh series, Li 3 HS has the lowest Ch-BVS value of –1.44, which is higher than that for Na 3 HSe (–1.32). Since we have estimated r(H – ) for each compound (Fig. 3b ), we can redefine the tolerance factor ( t ’) (see Supplementary Table 6 ). It is found that cubic hydride antiperovskites have large t ’ from 0.93 to 0.99, while orthorhombic Na 3 HS has t ’ = 0.85. The redefined t ’ for Li 3 HCh is closer to unity and has a narrower range. For example, Li 3 HS with a minimum t of 0.85 changes to t ’ = 0.95 when the observed r(H – ) is applied. Therein lies the extraordinary size flexibility of hydride, that is, the marked variation in bond length of H–Li in HLi 6 octahedra, from a maximum of 2.11 Å for Li 3 HTe to a minimum of 1.93 Å for Li 3 HS, as shown in Fig. 3d . The obtained bond-length difference of 0.09 Å for hydride antiperovskites is much larger than those of other antiperovskites with B = N (0.04 Å), O (0.03 Å), and F (0.01 Å). However, from a broader perspective, antiperovskites generally have larger octahedral size variations than conventional oxide perovskites, developing the potential to tailor structures toward acquiring new functions. Until now, we had a sharp picture of the large size variation of hydride anion. The chalcogenide anion, however, is also polarizable. To critically evaluate the role of anions in stabilizing the cubic structure, we estimated the radius of each ion using Bader population analysis, which partitions the first-principles-calculated charge density grid into the Bader region of each ion (see Methods in Supplementary Information) [44] . The resulting Bader radius of Li + only increases from 0.94 to 0.97 Å when the A-site chalcogenide anion increase from S 2– to Te 2– , whereas the Bader radius of H – ion expands from 1.38 to 1.48 Å (Supplementary Table 7 ). The large size variation of H – is also evidenced in Na 3 HCh. Interestingly, the change in Bader radius of Ch 2– ions is comparable to that of H – ions; the Bader radii of Se 2– and H – are 2.06 and 1.42 Å, respectively, in Li 3 HSe and increase to 2.24 and 1.52 Å in Na 3 HSe. However, when applying the external pressure (5 GPa) to M 3 HCh, the Bader radius of H – decreases more substantially than that of Ch 2– (Supplementary Fig. 11 ). The hydride ion is more sensitive to the applied pressure than chalcogenide. Given that most of M 3 HCh compounds are currently synthesized by high pressure, we argue that the flexible hydride is more critical for stabilizing the cubic symmetry. To investigate the thermodynamic stability of this series of hydride antiperovskites, we evaluated the formation enthalpy Δ H of M 3 HCh (M = Li, Na) in the reaction (MH + M 2 Ch → M 3 HCh) under 0 and 5 GPa based on first-principles calculations, where Δ H is defined as Δ H = H (M 3 HCh) − { H (M 2 Ch) + H (MH)}. Calculations showed that Li 3 HS, Na 3 HS, and Na 3 HSe are thermodynamically unstable at 0 GPa (Δ H > 0), but are stabilized under high pressure (Fig. 4a ). On the other hand, Li 3 HTe and Na 3 HTe with large t ’ values (0.99 and 0.96, respectively) are stable even at ambient pressure. Hence, the proof-of-concept trial to synthesize Na 3 HTe was conducted by heating a mixed pellet of NaH and Na 2 Te at 400 °C overnight in a vacuum-sealed Pyrex tube. The resulting SXRD pattern (Supplementary Fig. 12 ) yielded a cubic phase with a = 4.76717(5) Å, which is identical with the sample obtained under high pressure ( a = 4.76349(2) Å) and antisite anion disorder exists in neither case (Supplementary Table 8 ). In addition, the Gibbs free energy difference (Δ G ) showed that Li 3 HSe is stable at ambient pressure (Δ G = −0.01 eV/f.u. ), despite the slightly positive value of Δ H (Fig. 4a ); our preliminary synthesis under simple ambient conditions has failed, but there remains room for adjusting parameters, such as partial H 2 gas pressure. Fig. 4: Formation enthalpy and phonon calculations. a Formation enthalpy Δ H in the reaction MH + M 2 Ch → M 3 HCh (M = Li, Na) under 0 and 5 GPa. b Phonon band structures and partial phonon density of states (DOS) of Li, H, and S atoms in Li 3 HS under 0 GPa and c 5 GPa. The negative number of the vertical axis represents imaginary frequency. d HM 6 octahedral rotation associated with the phonon mode denoted by yellow circles in phonon band dispersion, where ω rot is the frequency of the HM 6 rotational mode at M point. e Displacement ellipsoids of Li atoms depicted at 50% probability level obtained from Rietveld refinement of ND in Li 3 HS. Full size image Electron and phonon calculations The electronic band structures at 0 GPa (Supplementary Fig. 13 ) obtained using first-principles calculations show that all the compounds have relatively large bandgaps: 4.2 eV for Li 3 HS, 3.5 eV for Li 3 HSe, 2.9 eV for Li 3 HTe, 2.9 eV for Na 3 HS, 2.8 eV for Na 3 HSe and 2.7 eV for Na 3 HTe. Although GGA-PBE exchange-correlation functional generally underestimates bandgaps [45] , our compounds are expected to have electronically good insulating properties to meet the requirements as a solid electrolyte. Phonon band structures of the hydride antiperovskites at 0 and 5 GPa were calculated using lattice dynamics within harmonic approximation (see Fig. 4b, c for Li 3 HS and Supplementary Fig. 14 for the others), including the hypothetical cubic c-Na 3 HS. All the synthesized cubic compounds are found to be dynamically stable at 5 GPa. In contrast, the c-Na 3 HS under 0 and 5 GPa exhibits imaginary phonon modes at the M and R points, corresponding to in-phase and out-of-phase rotations of the HM 6 octahedral rotation, respectively [46] , which as a result confirms the experimentally observed orthorhombic structure o-Na 3 HS with the a + b – b – tilting in Glazer notation. Li 3 HSe, Li 3 HTe, and Na 3 HTe are dynamically stable even at 0 GPa without any imaginary phonon frequencies. For Li 3 HS and Na 3 HSe (dynamically stable at 5 GPa), imaginary phonon modes (lattice instabilities) appear at M and R points under 0 GPa, which is inconsistent with experimental observations of the cubic phase after quenching from 5 GPa; this inconsistency might be resolved by including anharmonic effects of phonons at finite temperatures, which is the case of cubic SrTiO 3 [47] . The calculated phonon dispersions of M 3 HCh (M = Li, Na) and atom-projected phonon DOS are quite unique; high frequencies associated with optical phonons are ascribed to local vibrations of the lighter H – ion, whereas vibrations by heavier M + and Ch 2– ions are responsible for low phonon frequencies, along with relatively flat dispersions. Furthermore, the phonon band center of M + ions decreases as the Ch 2– ion becomes larger (e.g., 9.6 to 9.2 to 8.4 THz for Li 3 HCh), suggesting a tunability of lattice softness for mobile M + ions. Given the concept of “the softer the lattice, the better” [18] , [20] , [21] , [23] , [25] , [31] and the relatively large calculated bandgap, M 3 HCh antiperovskites should be a promising candidate as Li/Na solid-state electrolytes. In the next section, we will explore ionic transport properties in this series of hydride-based antiperovskites from a theoretical and experimental point of view. Ionic conductivity Nudged elastic band (NEB) calculations were used to estimate the energy barrier for cationic transport. Previous studies on Li 3 OCl proposed two transport mechanisms, i.e., Li hopping via vacancy mechanism and Li interstitial dumbbell hopping along edges of LiO 6 octahedra [10] , [12] . We calculated migration barriers for Li/Na transport in M 3 HCh based on these two mechanisms, and the results are displayed in Fig. 5a for the vacancy mechanism and Fig. 5b for the dumbbell mechanism. The energy barriers via vacancy mechanism range from 0.15 eV (o-Na 3 HS, Supplementary Fig. 15 ) to 0.32 eV (Li 3 HTe), while the dumbbell mechanism has a much smaller energy barrier from 0.05 eV (Na 3 HSe) to 0.14 eV (Li 3 HTe). The calculated energy barriers via both of mechanisms for M 3 HCh are notably low, and the difference of more than half between two mechanisms is also observed in previously reported antiperovskites (e.g., in Li 3 OCl, 0.31 eV and 0.15 eV for vacancy and dumbbell mechanisms, respectively) [12] . It should also be noted that the calculated migration barrier (3.49 eV) for hydride (H – ) hopping via vacancy in Li 3 HS (Supplementary Fig. 16 ) is much higher than that of Li + (0.20 eV), indicating that H – anions hardly migrate in our antiperovskite. From the results of potentiostatic measurement of the symmetric cell Li 3 PS 4 /Li 2.9 H(S 0.9 I 0.1 )/Li 3 PS 4 , the steady-state current suggesting the sole motion of Li + in iodine-doped Li 3 HS is observed in Supplementary Fig. 17 . Fig. 5: Ionic conductivities of M 3 HCh antiperovskites (M = Li, Na, and Ch = S, Se, Te). Low-barrier migration pathways for a vacancy and b interstitial dumbbell migration in M 3 HCh. Top-left insets show M + migration when viewing HM 6 octahedron from the top to down. For orthorhombic Na 3 HS, there are many migration pathways, one of which is shown as a representative example (see Supplementary Fig. 15 for details). c Migration barriers for cation transport via the vacancy and interstitial dumbbell mechanism in M 3 HCh as a function of the force constant k rot with respect to the HM 6 rotational motion. d Arrhenius plots of the total conductivity values for undoped M 3 HCh cold-pressed samples in the temperature range from 25 to 100 °C. Full size image To our surprise, the energy barrier is largest for Ch = Te, followed by Se and S. This seems counterintuitive since the cell volume increases (corresponding to the widening of the channels for Li/Na transport) as the ionic radius of chalcogenide ion increase from S to Se and then Te. At the same time, the phonon band center of Li/Na becomes lower (enhancing the softness of lattice), which implies that other factors such as local lattice dynamics are playing a role in ion diffusion. A systematic investigation of phonon dispersions in M 3 HCh revealed that the rotational motion of the HM 6 octahedron reflecting on the phonon mode at M point (Fig. 4d ) is essential to understand the unusual Ch dependence. This rotational motion corresponds well to the migration direction of M + ions to adjacent sites and displacement ellipsoids (anisotropic atomic displacement parameters) of Li/Na (Fig. 4e ) obtained from the Rietveld refinement conform well to the rotational mode. The frequency of this phonon mode, ω rot , decreases with decreasing the Ch 2– size (1.4 i , 3.7 and 5.7 THz for Li 3 HS, Li 3 HSe and Li 3 HTe and 0.6 i and 2.1 THz for Na 3 HSe and Na 3 HTe), demonstrating the softening of this specific rotational phonon. For both Li/Na migration mechanism, ω rot 2 · m M (where m M is the atomic mass of M), which corresponds to the force constant k rot with respect to the rotational motion, exhibits a positive linear correlation with energy barriers (Fig. 5c ). The decreasing trend of ω rot for Te → Se → S is directly related to the dynamic stability or the phase transition between the cubic phase and the tilted orthorhombic phase (Fig. 4 and Supplementary Fig. 14 ). Thus, the softening of M + ion migration (or octahedral rotational) mode could be the origin of the low energy migration energy of hydride antiperovskites. Experimentally, we measured lithium/sodium-ion conductivity of cold-pressed M 3 HCh samples (M = Li, Na; Ch = S, Se, Te) using electrochemical impedance spectroscopy (EIS). As a representative example, we show in Supplementary Fig. 18 Nyquist plots of Na 3 HSe, featuring typical ionic impedance response with a semicircle which has a capacitance of ~10 –10 F at high frequencies and a low-frequency tail. Since the bulk and grain boundary resistance cannot be specifically deconvoluted [48] , the total conductivity in Fig. 5d is attributed to the bulk and grain boundary resistance, which might be the reason why no clear trend in the composition dependence of ionic conductivity is observed. The activation energies obtained from the Arrhenius fit for the pristine M 3 HCh (Fig. 5d ) are in the range of 0.44 to 0.53 eV for cubic phases and 0.30 eV for orthorhombic Na 3 HS, which are comparable with other superionic conductors such as garnet Li 7 La 3 Nb 2 O 12 [49] and β-Li 3 PS 4 [50] . Compared with the computed migration barrier (Fig. 5a, b ), the experimentally obtained activation energy (Fig. 5d ) is relatively large. The discrepancy might result from two facts: the low concentration of intrinsic charge carriers (i.e., vacancies/interstitials) which we expect in the synthesized sample, whereas the calculated migration barriers assume intrinsic vacancies or interstitials of lithium/sodium. In addition, the migration barrier is separate from defect formation energy (which we list in Supplementary Table 9 ), whereas they are reflected in the experimental activation energies. Moreover, the computed compositional dependence (Fig. 5c ) is not observed, probably due to the non-negligible resistive grain boundary and interfacial impacts on the conductivity measurement [51] . Here, we take the cubic Na 3 HSe compound as an example to fulfill the potential of the deformable anion matrix for fast sodium ionic diffusion. When creating a small number of sodium vacancies in Na 2.9 H(Se 0.9 I 0.1 ), the total ionic conductivity increased to ~1 × 10 –4 S/cm at 100 °C with two orders of magnitude higher than the undoped one (Fig. 6a ). It is also noteworthy that the Nyquist plots of I-doped Na 2.9 H(Se 0.9 I 0.1 ) sample at a lower temperature (Supplementary Fig. 19 ) show two semicircles at the high frequency where the small half-semicircle corresponds to the grain/bulk resistance and a low-frequency tail. As shown in Fig. 6b , the bulk activation energy for sodium-ion transport in Na 2.9 H(Se 0.9 I 0.1 ) is determined as E a,bulk = 0.18 eV, which is close to the calculated migration barrier of 0.16 eV via vacancy mechanism in Na 3 HSe (Fig. 5a ). Detailed structural characterization of Na 2.9 H(Se 0.9 I 0.1 ) is shown in Supplementary Fig. 20 and Supplementary Table 10 . Fig. 6: Na + diffusion in Na 3 HSe and Na 2.9 H(Se 0.9 I 0.1 ). a Impedance plots at 100 °C of the cold-pressed pellets and the impedance is normalized to the respective pellet thickness. b Arrhenius plots of the total conductivity (circles) and bulk conductivity (triangles). c 23 Na static NMR spectra measured under 7 T at room temperature. For Na 2.9 H(Se 0.9 I 0.1 ), observed spectra (black solid), fitting spectra (red dashed), and deconvolved peak 1 with C Q = 1.30 MHz, ŋ = 0.16 (green) and peak 2 with C Q = 1.33 MHz, ŋ = 0.03 (blue). Full size image The 23 Na NMR data (Fig. 6c ) exhibit a distinct behavior associated with the bulk diffusion of Na + ions in pristine and I-doped samples. The analysis of the spectra revealed that quadrupole interaction is dominant in Na 2.9 H(Se 0.9 I 0.1 ) reflecting the faster Na + diffusion, whereas dipole–dipole interactions of the 23 Na nuclei are non-averaged in the isostructural Na 3 HSe, Na 3 HTe, and I-doped variant [52] . The line width of iodine-doped sample is narrower than that of undoped one, implying that faster short-range (i.e., bulk) ion dynamics. Furthermore, the line widths of Na 3 HTe NMR spectra (Supplementary Fig. 21 ) were observed to decrease with increasing temperature (known as motional narrowing) and dipole–dipole interactions are progressively averaged due to the thermally activated motion of the Na ions [21] . The enhancement of Na + conductivity we have achieved by the common aliovalent substitution approach promises the excellent potential of soft hydride–chalcogenide anion framework for Li + /Na + diffusion. There is still much room for improvement, such as mixed halide doping in A and/or B site, in future owing to the versatility of the perovskite-based crystal structures. By exploiting the simple but unique hydride anion, a series of antiperovskites with the formula of M 3 HCh (M = Li, Na; Ch = S, Se, Te) has been successfully synthesized. Detailed structural characterizations demonstrate that the highly flexible size of hydride in the octahedral center explains the robustness of the ideal cubic structure in a wide compositional range with a 0.09 Å H–M bond difference, much longer than other antiperovskites and perovskites. Theoretically, the family of LiRAPs and NaRAPs composed by soft anion sublattices of polarizable hydride and chalcogenide are shown to have low migration barriers for Li/Na bulk transport, where the rotational phonon mode by HM 6 octahedron possibly facilitates the Li/Na migration. Experimentally, high conductivity and low bulk activation energy have been demonstrated in the iodine-doped Na 2.9 H(Se 0.9 I 0.1 ), with the total ionic conductivity of 1 × 10 –4 S/cm at 100 °C. Further optimization through structural design and chemical doping would promise to achieve their full potential. The exploitation of size-flexible hydride anion developed in this work will be favorable for other ion-conducting materials, also help to induce novel states of matter and excitation phenomena. Materials synthesis Polycrystalline M 3 HCh samples (M = Li, Na; Ch = S, Se, Te) were synthesized via high-pressure solid-state reactions using MH and M 2 Ch as starting reagents. We used as-received LiH (Sigma-Aldrich, 99%), Li 2 S (Sigma-Aldrich, 99%), NaH (Sigma-Aldrich, 99%), Na 2 S (Sigma-Aldrich, 99%), Na 2 Se (Kojundo, 99%), Na 2 Te (Kojundo, 99%), while Li 2 Se and Li 2 Te were prepared using LiEt 3 BH (Sigma-Aldrich), Se (Rare Metallic Co., LTD., 99.9%) and Te (Rare Metallic Co., LTD., 99.9%). There is a tendency that excess use of alkali metal hydride improves sample purity. The starting materials were well-ground and pelletized, and the pellets were inserted into a boron nitride (BN) sleeve. The two ends of the sleeve were then sealed with BN caps. The assemble was loaded into a graphite tube heater and then enclosed in a pyrophyllite cube serving as a pressure medium. All above procedures were handled in a N 2 -filled glovebox due to air and moisture sensitivity of the precursors and synthesized materials. Finally, the assembly was pressed at 5 GPa, heated to 700 °C in 10 min, kept for 2 h, and cooled down to room temperature in 5 min before pressure was released. All the iodine-doped samples (e.g., Na 2.9 H(Se 0.9 I 0.1 ), Na 2.9 H(Te 0.9 I 0.1 ), Li 2.9 H(S 0.9 I 0.1 )) were successfully synthesized using NaI/LiI (Sigma-Aldrich, 99%) as iodine source under the same condition with undoped one. Powder X-ray and neutron diffraction We characterized the purity and crystal structures of as-prepared M 3 HCh samples at room temperature by powder X-ray diffraction (XRD) measurements using Rigaku Smart Lab with Cu radiation and Bruker D8 ADVANCE with Mo radiation. High-resolution synchrotron XRD experiments (SXRD) were performed at BL02B2 of SPring-8 (Japan) equipped with MYTHEN solid-state detectors. Time-of-flight(TOF) powder neutron diffraction (ND) data of Li 3 HS and Na 3 HS samples were collected on iMATERIA and SPICA diffractometers installed at the Material and Life science Facility (MLF) in the Japan Proton Accelerator Research Complex (J-PARC). The powder samples were sealed in cylindrical vanadium cells of dimensions 6 mm in diameter, 55 mm in height, and 100 μm in thickness. Rietveld refinements were performed on neutron data taken at the backscattering bank (2 θ = 155° for iMATERIA and 2 θ = 160.77° for SPICA). Data were evaluated and refined using the FULLPROF suite, JANA2006, and Z-Rietveld softwares [53] . VESTA was used to display crystal structure and to calculate geometric properties. Impedance spectroscopy Ionic conductivities of cold-pressed pellets of M 3 HCh were measured by electrochemical impedance spectroscopy (EIS) with a constant voltage of 10 mV in the frequency range of 1 MHz to 0.1 Hz using an ECS Modulab potentiostat/galvanostat. Around 80 mg of the specimen was placed between two stainless-steel rods as an ion-blocking electrode in a custom-made Swagelok cell and pressed into a 10 mm diameter pellet by a hydraulic press at 18 MPa for 1 min in an Ar-filled glovebox. For activation energy measurements, we applied a temperature loop starting from 25 °C to 100 °C. The measurements at each temperature were collected after being held for 3 h to ensure the temperature stabilization. All equivalent circuits of Nquist plots were fitted using the EC-Lab software package Z-fit. NMR spectroscopy 23 Na NMR measurements were performed using JNM-ECA300 under 7 T with the 23 Na Lamor frequency of 79.5 MHz and ECA600 (JEOL) under 14 T with 158.8 MHz frequency. For magic-angle spinning (MAS) NMR, the sample was packed into a 4-mm zirconia rotor in an Ar-filled glovebox and the spinning speed was 10 kHz. For variable-temperature 23 Na static NMR, the sample was sealed in an evacuated borosilicate glass tube. The 23 Na chemical shifts of all spectra were referenced to 1 M NaCl aqueous solution at 0 ppm and the peaks of the spectra were deconvoluted using a Dmfit program. To assign the observed 23 Na spectra, first-principles calculations based on DFT were carried out using the WIEN2k codes [54] , [55] . The muffin-tin radius, R MT , of Na, H, and Se atoms was 2.0, 1.5, and 2.0, respectively, for cubic Na 3 HSe. The volume optimization was performed prior to the chemical shift calculation. Self-consistent cycles were carried out at an energy convergence of 0.0001 Ry. The R MT K max determining the number of basis function was set to 7.0, G max was 12, and the number of k -points in the irreducible Brillouin zone was 35. The electric-field gradient (EFG), the asymmetry parameter ( ŋ ), and the magnetic shielding coefficient ( σ iso ) were calculated for the final optimized structure. To convert σ iso into the chemical shift ( δ iso ) for comparison, σ iso of Na 2 SiO 3 with δ iso = 20.0 ppm [56] , α-Na 2 Si 2 O 5 with δ iso = 17.4 ppm [52] , and Na 2 SO 4 with δ iso = –8.5 ppm [52] were calculated in the same manner.